An isoform of retinoid-related orphan receptor β directs differentiation of retinal amacrine and horizontal interneurons Amacrine and horizontal interneurons integrate visual information as it is relayed through the retina from the photoreceptors to the ganglion cells. The early steps that generate these interneuron networks remain unclear. Here we show that a distinct retinoid-related orphan nuclear receptor β1 (RORβ1) isoform encoded by the retinoid-related orphan nuclear receptor β gene ( Rorb ) is critical for both amacrine and horizontal cell differentiation in mice. A fluorescent protein cassette targeted into Rorb revealed RORβ1 as a novel marker of immature amacrine and horizontal cells and of undifferentiated, dividing progenitor cells. RORβ1-deficient mice lose expression of pancreas-specific transcription factor 1a (Ptf1a) but retain forkhead box n4 factor (Foxn4), two early-acting factors necessary for amacrine and horizontal cell generation. RORβ1 and Foxn4 synergistically induce Ptf1a expression, suggesting a central role for RORβ1 in a transcriptional hierarchy that directs this interneuron differentiation pathway. Moreover, ectopic RORβ1 expression in neonatal retina promotes amacrine cell differentiation. Amacrine and horizontal cells integrate visual information as it is relayed through the retinal layers from the light-sensitive photoreceptors to the ganglion cells that form the optic nerve. Horizontal cells modify synaptic transmission between photoreceptors and bipolar cells whereas amacrine cells modify transmission between bipolar and ganglion cells [1] . These inhibitory interneuron networks are critical for visual function but the controls that generate amacrine and horizontal cells are incompletely understood. The different cell types of the neural retina are derived from multipotent progenitor cells [2] , [3] , [4] , [5] . Transcription factors in dividing progenitor cells or in newly post-mitotic precursor cells often determine retinal cell differentiation fates [6] , [7] , [8] . The forkhead box factor forkhead box n4 factor (Foxn4) and the basic helix-loop-helix (bHLH) factor pancreas-specific transcription factor 1a (Ptf1a) are required for differentiation of both horizontal and amacrine cells in mice, suggesting that a common transcriptional signal induces the formation of both interneuron classes [9] , [10] , [11] . The nature of this initial stimulus is unclear but Foxn4 expression in progenitor cells is succeeded by Ptf1a expression in post-mitotic precursor cells [9] , [10] , [11] , [12] , [13] , suggesting the involvement of a transcriptional hierarchy. In addition, the homeodomain protein Prox1 is required for horizontal cell differentiation [14] , whereas bHLH proteins Neurod1 (Nd1) and Neurod4 (Nd4, or Math3) are required for amacrine cell differentiation [15] , suggesting that other controls promote divergence of amacrine and horizontal cell lineages. Other transcription factors of the bHLH [16] , [17] , [18] , non-basic HLH [19] , homeodomain [20] , [21] , [22] and other families [23] , [24] , [25] further influence diversity in amacrine cell sub-lineages. The retinoid-related orphan nuclear receptor β gene ( Rorb , Nr1f2 ) mediates several neurodevelopmental functions. A total Rorb deletion impaired circadian behaviour, hindlimb motor control [26] , opsin induction in cone photoreceptors [27] and differentiation of rod photoreceptors [28] . The means by which developmental genes such as Rorb are able to control diverse cellular functions are often unclear. Rorb encodes two N-terminal isoforms, RORβ1 and RORβ2, with undefined functions [29] . Here, we report a key role for RORβ1 in amacrine and horizontal cell differentiation. Moreover, RORβ1 and Foxn4 synergistically activate the Ptf1a gene, suggesting that cooperation between this orphan receptor isoform and Foxn4 stimulates amacrine and horizontal cell generation. Differential expression of RORβ1 and RORβ2 isoforms To investigate specific functions for the isoforms encoded by Rorb , we analysed the expression of RORβ1 and RORβ2 mRNA during retinal development in mice ( Fig. 1a ). RORβ1 mRNA displayed a broad peak between mid-embryonic stages and the first postnatal week. RORβ1 mRNA expression then declined and was maintained at lower levels into adulthood. In contrast, RORβ2 mRNA was first detected at late embryonic stages and displayed a prominent rise over the first postnatal week. These contrasting expression profiles suggested that each isoform mediates specific functions in retinal development with RORβ1 serving a unique role at earlier stages of neurogenesis. 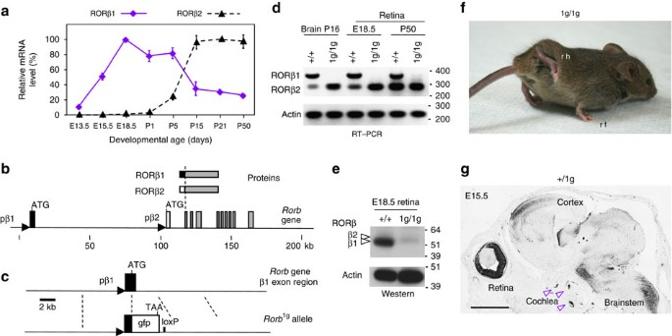Figure 1: Differential expression of RORβ isoforms and targeted deletion of RORβ1. (a) RORβ1 and RORβ2 mRNA expression profiles in mouse retinal development, determined by qPCR analysis. Levels for each isoform are indicated as percentages relative to the highest level, assigned a value of 100%. (b)Rorbgene with RORβ1- and RORβ2-specific exons depicted as black and white boxes, respectively, common exons as grey boxes and RORβ1 and RORβ2 promoter regions as triangles. (c) Targeted replacement of the coding portion of the RORβ1-specific exon with a gfp cassette that carries a TAA translational stop codon. Excision of the neomycin-resistance ACN cassette left a residual loxP site in theRorb1gallele. (d) Loss of RORβ1 mRNA and retention of RORβ2 mRNA in brain and retina in 1g/1g mice shown by PCR with control analysis for β-actin. DNA size marker, bp. (e) Loss of RORβ1 protein in the retina in 1g/1g mice shown on a western blot with control analysis for β-actin. Arrowheads, bands for RORβ1 (lower, ~52 kDa) and RORβ2 (upper, ~53 kDa). The gfp protein expressed in 1g/1g mice carries no RORβ protein sequence and was detected with antibody against gfp as a ~27-kDa band (not shown). Protein molecular size marker, kDa. (f) Abnormal gait in 1g/1g mice with exaggerated lifting and clasping of hindlimbs; rh, right hindlimb; rf, right forelimb. (g) Para-sagittal section of +/1g embryonic head showing gfp expression in retina, cochlea and brain. Expression of gfp was detected by immunohistochemistry (dark areas). Scale bar, 1 mm. Figure 1: Differential expression of RORβ isoforms and targeted deletion of RORβ1. ( a ) RORβ1 and RORβ2 mRNA expression profiles in mouse retinal development, determined by qPCR analysis. Levels for each isoform are indicated as percentages relative to the highest level, assigned a value of 100%. ( b ) Rorb gene with RORβ1- and RORβ2-specific exons depicted as black and white boxes, respectively, common exons as grey boxes and RORβ1 and RORβ2 promoter regions as triangles. ( c ) Targeted replacement of the coding portion of the RORβ1-specific exon with a gfp cassette that carries a TAA translational stop codon. Excision of the neomycin-resistance ACN cassette left a residual loxP site in the Rorb 1g allele. ( d ) Loss of RORβ1 mRNA and retention of RORβ2 mRNA in brain and retina in 1g/1g mice shown by PCR with control analysis for β-actin. DNA size marker, bp. ( e ) Loss of RORβ1 protein in the retina in 1g/1g mice shown on a western blot with control analysis for β-actin. Arrowheads, bands for RORβ1 (lower, ~52 kDa) and RORβ2 (upper, ~53 kDa). The gfp protein expressed in 1g/1g mice carries no RORβ protein sequence and was detected with antibody against gfp as a ~27-kDa band (not shown). Protein molecular size marker, kDa. ( f ) Abnormal gait in 1g/1g mice with exaggerated lifting and clasping of hindlimbs; rh, right hindlimb; rf, right forelimb. ( g ) Para-sagittal section of +/1g embryonic head showing gfp expression in retina, cochlea and brain. Expression of gfp was detected by immunohistochemistry (dark areas). Scale bar, 1 mm. Full size image Deletion of the RORβ1 isoform To determine the role of RORβ1 and to facilitate detection of its expression at the cellular level, we replaced the RORβ1-specific exon with a green fluorescent protein (gfp) cassette in mice. RORβ1 and RORβ2 are identical in their central DNA-binding and C-terminal domains but differ in their N-terminal extensions, consisting of 2 and 13 amino acids, respectively ( Fig. 1b ). RORβ1 and RORβ2 are expressed from distinct promoters upstream of their respective 5′-coding exons in the Rorb gene. The gfp cassette was inserted by targeted mutagenesis in embryonic stem cells, which were used to generate mice carrying this Rorb 1g allele ( Fig. 1c ). Southern blot and genomic sequencing analyses confirmed the structure of the Rorb 1g allele. RORβ1-specific mRNA was undetectable, whereas RORβ2-specific mRNA remained intact in the brain and retina of homozygous Rorb 1g/1g (1g/1g) mice ( Fig. 1d ). Western blot analyses demonstrated loss of the major RORβ1-specific protein band and retention of the minor, RORβ2-specific band in the retina of 1g/1g embryos ( Fig. 1e ). Heterozygous +/1g mice showed no overt phenotype but 1g/1g mice displayed abnormal gait with exaggerated raising of the hindlimbs similar to that described for Rorb −/− mice lacking all RORβ isoforms [26] , indicating that the RORβ1 isoform is critical for hindlimb motor control ( Fig. 1f ). Retinal expression pattern of Rorb 1g allele RORβ1 expression was traced in +/1g mice, which revealed gfp expression in the embryonic retina as well as in the immature cochlea, brainstem, spinal cord and cerebral cortex, shown at embryonic day 15.5 (E15.5) in Fig. 1g . In the retina, gfp expression displayed a dynamically changing pattern beginning in neuroblastic cells as early as E11.5. Strong gfp signals were detected in the nascent amacrine cell zones in both the inner nuclear layer (INL) and ganglion cell layer during the embryonic and neonatal period when amacrine cells are generated [5] ( Fig. 2a ). By postnatal day 7 (P7), gfp was also detected within the inner plexiform synaptic layer in two stratified layers characteristic of the lateral projections of amacrine cells. Developmentally changing but weaker gfp signals were also detected in bipolar neurons, photoreceptors and Muller glia. In general, gfp signals declined after P7 with low levels remaining at older stages, consistent with previous data for Rorb mRNA [30] , [27] . In the embryonic retina, many gfp + cells in the outer neuroblastic layer were positive for proliferating cell nuclear antigen (PCNA), a marker of dividing progenitor cells in G1, S and G2 phases of the cell cycle [31] ( Fig. 2b ). 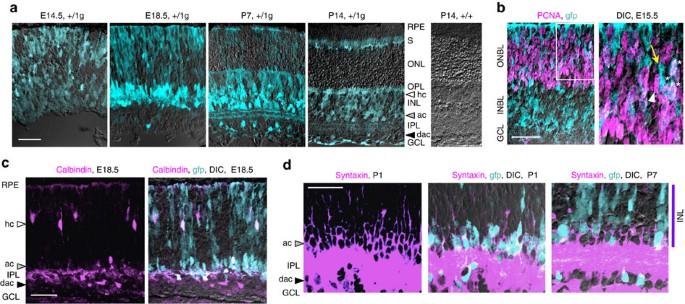Figure 2: Expression ofRorb1gallele in retina. (a) Developmental analysis in +/1g mice showing gfp (turquoise fluorescence) overlaid on differential interference contrast (DIC) images to show cell layers. GCL, ganglion cell layer, INL, inner nuclear layer, IPL, inner plexiform layer, ONL, outer nuclear layer, OPL, outer plexiform layer, RPE, retinal pigmented epithelium, S, inner/outer segment layers. White, grey and black arrowheads indicate horizontal cell (hc), amacrine cell (ac) and displaced amacrine cell (dac) zones, respectively. Control +/+ retina shows absence of gfp signal. Scale bar, 30 μm in all panels. (b) Detection of proliferative progenitor cells (PCNA, purple) that express gfp (turquoise) overlaid on a DIC image in a +/1g embryo. Double detection of gfp and PCNA required HCl pre-treatment of sections. In the outer neuroblastic layer (ONBL), many cells co-express both PCNA and gfp (white or whitish). Right, enlargement of boxed ONBL area showing PCNA+/gfp+cells (asterisks), PCNA+cells (white arrowhead) and gfp+cells (yellow arrow). (c)Rorb1gexpression (turquoise) in immature horizontal, amacrine and displaced amacrine cells identified with calbindin (purple) in a +/1g embryo. Co-localization of calbindin and gfp results in whitish cells, overlaid on a DIC image. (d)Rorb1gexpression (turquoise, soma) in immature amacrine cells identified with syntaxin (purple, honeycomb pattern around the soma). At P1 (left two panels), most syntaxin+cells are gfp+but at P7 (right), fewer are gfp+ and many have only weak gfp signals. Amacrine cells form a zone ~3 soma deep in the INL. Figure 2: Expression of Rorb 1g allele in retina. ( a ) Developmental analysis in +/1g mice showing gfp (turquoise fluorescence) overlaid on differential interference contrast (DIC) images to show cell layers. GCL, ganglion cell layer, INL, inner nuclear layer, IPL, inner plexiform layer, ONL, outer nuclear layer, OPL, outer plexiform layer, RPE, retinal pigmented epithelium, S, inner/outer segment layers. White, grey and black arrowheads indicate horizontal cell (hc), amacrine cell (ac) and displaced amacrine cell (dac) zones, respectively. Control +/+ retina shows absence of gfp signal. Scale bar, 30 μm in all panels. ( b ) Detection of proliferative progenitor cells (PCNA, purple) that express gfp (turquoise) overlaid on a DIC image in a +/1g embryo. Double detection of gfp and PCNA required HCl pre-treatment of sections. In the outer neuroblastic layer (ONBL), many cells co-express both PCNA and gfp (white or whitish). Right, enlargement of boxed ONBL area showing PCNA + /gfp + cells (asterisks), PCNA + cells (white arrowhead) and gfp + cells (yellow arrow). ( c ) Rorb 1g expression (turquoise) in immature horizontal, amacrine and displaced amacrine cells identified with calbindin (purple) in a +/1g embryo. Co-localization of calbindin and gfp results in whitish cells, overlaid on a DIC image. ( d ) Rorb 1g expression (turquoise, soma) in immature amacrine cells identified with syntaxin (purple, honeycomb pattern around the soma). At P1 (left two panels), most syntaxin + cells are gfp + but at P7 (right), fewer are gfp+ and many have only weak gfp signals. Amacrine cells form a zone ~3 soma deep in the INL. Full size image Further analysis co-localized gfp signals with calbindin, a marker of horizontal cells and a sub-population of amacrine cells at late embryonic and neonatal stages ( Fig. 2c ). At early stages, almost all calbindin + horizontal cell precursors were gfp-positive. By P1, gfp was also detected in most cells that expressed syntaxin, a marker for all amacrine cell types ( Fig. 2d ). During later stages of differentiation, gfp signals declined in both calbindin + horizontal and syntaxin + amacrine cells. Thus, the data indicated that RORβ1 was expressed in progenitor cells and subsequently, at enhanced levels in newly generated horizontal and amacrine cell precursors, followed by declining levels during later development. Rorb 1g/1g mice lack amacrine and horizontal cells RORβ1-deficient mice displayed a collapsed inner plexiform layer, disorganized outer plexiform layer and a thin inner nuclear layer that was only 3 or 4 soma deep compared with ~6 soma deep in +/+ mice ( Fig. 3a ). These abnormalities reflected loss of horizontal and amacrine cells as demonstrated on retinal flatmounts analysed for calbindin, a marker of both cell classes ( Fig. 3b ). Ganglion cells were mis-located in the collapsed inner plexiform layer ( Fig. 3a ) but still formed an optic nerve in 1g/1g mice. Other major classes of retinal cells, including bipolar cells, Muller glia, rods and cones were present as indicated by histology and analysis of cell type markers ( Supplementary Fig. S1 ). 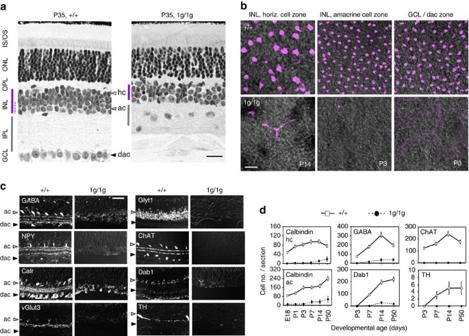Figure 3: Loss of amacrine and horizontal cells inRorb1g/1gmice. (a) Histological sections showing disorganized inner plexiform, outer plexiform and ganglion cell layers in 1g/1g mice at P35. Note the thin INL (purple bar) and mis-located ganglion cell soma in the collapsed IPL in 1g/1g mice. Amacrine cell zone in the INL is indicated by a dashed line in +/+ retina. Scale bar, 30 μm in all panels. (b) Retinal flatmounts analysed by confocal microscopy in the plane of horizontal (hc), amacrine (ac) and displaced amacrine (dac) cell zones using calbindin as a marker (purple) on DIC images to show tissue structure. Calbindin+horizontal and amacrine cells are missing in 1g/1g mice. (c) Retinal sections showing loss of representative amacrine cell markers (GABA, GlyT1, neuropeptide Y (NPY), ChAT, calretinin/calr, Dab1, vGlut3, TH) in 1g/1g mice at P14 (except NPY at P7). (d) Cell counts showing failure to generate amacrine and horizontal cells, identified with horizontal (calbindin/hc) and amacrine (calbindin/ac, GABA, ChAT, Dab1, TH) markers. Calbindin+horizontal and amacrine cells were distinguished in +/+ mice by morphology and location in the INL. Cell counts, given as mean±s.d., were based on analysis of 12 cryosections of the retina representing ≥3 mice at each age. Figure 3: Loss of amacrine and horizontal cells in Rorb 1g/1g mice. ( a ) Histological sections showing disorganized inner plexiform, outer plexiform and ganglion cell layers in 1g/1g mice at P35. Note the thin INL (purple bar) and mis-located ganglion cell soma in the collapsed IPL in 1g/1g mice. Amacrine cell zone in the INL is indicated by a dashed line in +/+ retina. Scale bar, 30 μm in all panels. ( b ) Retinal flatmounts analysed by confocal microscopy in the plane of horizontal (hc), amacrine (ac) and displaced amacrine (dac) cell zones using calbindin as a marker (purple) on DIC images to show tissue structure. Calbindin + horizontal and amacrine cells are missing in 1g/1g mice. ( c ) Retinal sections showing loss of representative amacrine cell markers (GABA, GlyT1, neuropeptide Y (NPY), ChAT, calretinin/calr, Dab1, vGlut3, TH) in 1g/1g mice at P14 (except NPY at P7). ( d ) Cell counts showing failure to generate amacrine and horizontal cells, identified with horizontal (calbindin/hc) and amacrine (calbindin/ac, GABA, ChAT, Dab1, TH) markers. Calbindin + horizontal and amacrine cells were distinguished in +/+ mice by morphology and location in the INL. Cell counts, given as mean±s.d., were based on analysis of 12 cryosections of the retina representing ≥3 mice at each age. Full size image Analysis of retinal sections ( Fig. 3c ) revealed loss of multiple amacrine cell sub-types in 1g/1g mice as indicated by loss of signals for: (i) γ-aminobutyric acid (GABA) and neuropeptide Y, markers of GABA-ergic cells, (ii) glycine transporter T1 (GlyT1) and disabled 1 (Dab1), markers of glycinergic cells, (iii) vesicular glutamate transporter 3 (vGlut3) a marker of glutamatergic cells, (iv) choline acetyl transferase (ChAT), a marker of cholinergic cells, (v) tyrosine hydroxylase (TH), a marker of dopaminergic cells, and (vi) calretinin (calr), a marker of ~40% of all amacrine cells of several sub-types. Analysis of pan-amacrine cell markers syntaxin 1 and Pax6 transcription factor confirmed a general depletion of amacrine cell types ( Supplementary Fig. S1 ). Counts of cells expressing representative amacrine (GABA, Dab1, ChAT, TH, calbindin) and horizontal (calbindin) markers revealed that amacrine and horizontal cells were missing from early stages of development in 1g/1g mice ( Fig. 3d ), indicative of a developmental failure to generate these cells rather than a later loss by degeneration. Expression of gfp was maintained in the retina in 1g/1g embryos, suggesting that progenitors continued to be generated in the absence of RORβ1 (not shown). Indeed, analysis of bromodeoxyuridine (BrdU) incorporation, an indicator of cell proliferation, revealed comparable numbers of BrdU + cells in +/+ and 1g/1g mice at E12.5 and P1 ( Fig. 4a ). Previous studies in Ptf1a -deficient mice showed that a lack of amacrine and horizontal cells was accompanied by an excess of ganglion cells, suggesting a possible fate switch for progenitors that normally would form amacrine and horizontal cells [10] , [11] . We similarly observed ~2-fold increased Brn3a + ganglion cell numbers at embryonic and neonatal ages in 1g/1g mice ( Fig. 4b ). During postnatal development, numbers of Brn3a + cells declined while increased numbers of caspase 3 + cells were detected in 1g/1g mice, suggesting that excess Brn3a + cells were subsequently lost by programmed cell death in 1g/1g mice. This phenotype of loss of horizontal and amacrine cells coupled with increased ganglion cell numbers, suggested that RORβ1, like Ptf1a, may influence a pathway with alternative differentiation outcomes of ganglion cell versus amacrine and horizontal cells [10] , [11] . 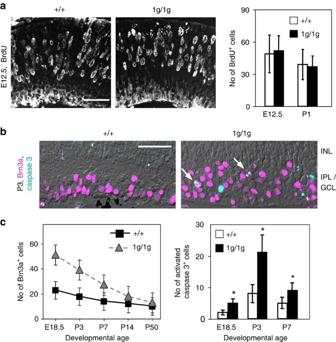Figure 4: Excess ganglion cells inRorb1g/1gmice. (a) Normal numbers of BrdU+proliferating cells were detected in the retina in 1g/1g mice 1 h after a pulse delivery of BrdU. Graph of BrdU+cell counts at E12.5 and P1 shows no differences between +/+ and 1g/1g mice; mean±s.d.;P>0.8. Counts represent BrdU+cells per 150 μm length of retina, determined on 10 μm thick cryosections. Scale bar, 30 μm in all panels. (b) Immunostaining for Brn3a+ganglion cells (purple) in retinal sections at P3. Sections were co-stained for activated caspase 3 (turquoise), a marker of apoptotic cells. Arrows, double-labelled cells in 1g/1g mice, which were rarely observed in +/+ mice. (c) The postnatal decline in excess Brn3a+cells correlated with increased cell death rates in 1g/1g mice. Left, counts of Brn3a+cells per 150 μm length of retina in 10 μm thick sections. For +/+ and 1g/1g differences at E18.5, P3 and P7,P<0.001. Right, counts of caspase 3+cells per section; mean±s.d.; *P<0.001. Statistical analyses were performed using Student’st-test. Figure 4: Excess ganglion cells in Rorb 1g/1g mice. ( a ) Normal numbers of BrdU + proliferating cells were detected in the retina in 1g/1g mice 1 h after a pulse delivery of BrdU. Graph of BrdU + cell counts at E12.5 and P1 shows no differences between +/+ and 1g/1g mice; mean±s.d. ; P >0.8. Counts represent BrdU + cells per 150 μm length of retina, determined on 10 μm thick cryosections. Scale bar, 30 μm in all panels. ( b ) Immunostaining for Brn3a + ganglion cells (purple) in retinal sections at P3. Sections were co-stained for activated caspase 3 (turquoise), a marker of apoptotic cells. Arrows, double-labelled cells in 1g/1g mice, which were rarely observed in +/+ mice. ( c ) The postnatal decline in excess Brn3a + cells correlated with increased cell death rates in 1g/1g mice. Left, counts of Brn3a + cells per 150 μm length of retina in 10 μm thick sections. For +/+ and 1g/1g differences at E18.5, P3 and P7, P <0.001. Right, counts of caspase 3 + cells per section; mean±s.d. ; * P <0.001. Statistical analyses were performed using Student’s t -test. Full size image Loss of transcription factor expression in Rorb 1g/1g mice The developmental stage at which RORβ1 acts relative to Foxn4, Ptf1a and other transcription factors involved in amacrine and horizontal cell differentiation was investigated. In situ hybridization detected the presence of Foxn4 but loss of Ptf1a mRNA in 1g/1g mice at E15.5 ( Fig. 5a ). Quantitative PCR (qPCR) analysis demonstrated a normal developmental profile for Foxn4 mRNA levels, whereas Ptf1a mRNA was lacking from early stages in 1g/1g mice ( Fig. 5b ). Previously, a partial loss of Nd1 and Nd4 mRNA was reported in Foxn4 −/− mice at E15 [9] , [32] . In situ hybridization revealed a moderate reduction of Nd1 and Nd4 mRNA signals in 1g/1g embryos ( Fig. 5a ) and qPCR revealed 37±5 and 45±8% ( P <0.001) decreases of Nd1 and Nd4 mRNA levels, respectively, in 1g/1g embryos at E14.5 ( Supplementary Fig. S2 ). 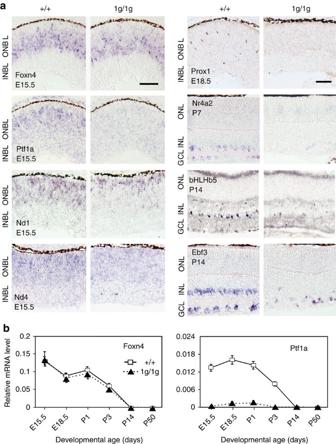Figure 5: Expression of retinal transcription factors inRorb1g/1gmice. (a) Transcription factor expression analysed byin situhybridization (Foxn4, Ptf1a, Nd1, Nd4, Nr4a2, Ebf3) or immunohistochemistry (Prox1, bHLHb5), at stages when each factor normally displays prominent expression (early stages, left, or later maturation stages, right). Ptf1a was overtly and Nd1 and Nd4 were modestly reduced in 1g/1g mice. Expression of horizontal (Prox1) and amacrine sub-lineage (Nr4a2, bHLHb5, Ebf3) markers was severely reduced in 1g/1g mice. Scale bar, 30 μm. (b) qPCR analysis demonstrating normalFoxn4but reducedPtf1amRNA levels inRorb1g/1gmice during development. Each point represents mean of three analyses on pooled retina (>4 mice) at each age. Plots based on mean±s.d. at each age. Figure 5: Expression of retinal transcription factors in Rorb 1g/1g mice. ( a ) Transcription factor expression analysed by in situ hybridization (Foxn4, Ptf1a, Nd1, Nd4, Nr4a2, Ebf3) or immunohistochemistry (Prox1, bHLHb5), at stages when each factor normally displays prominent expression (early stages, left, or later maturation stages, right). Ptf1a was overtly and Nd1 and Nd4 were modestly reduced in 1g/1g mice. Expression of horizontal (Prox1) and amacrine sub-lineage (Nr4a2, bHLHb5, Ebf3) markers was severely reduced in 1g/1g mice. Scale bar, 30 μm. ( b ) qPCR analysis demonstrating normal Foxn4 but reduced Ptf1a mRNA levels in Rorb 1g/1g mice during development. Each point represents mean of three analyses on pooled retina (>4 mice) at each age. Plots based on mean±s.d. at each age. Full size image Loss or reduced expression of transcription factors that influence specifically horizontal (Prox1, Lim1) or amacrine (Nr4a2, bHLHb5, Ebf3) sub-lineage differentiation was also detected in 1g/1g mice by in situ hybridization, immunohistochemical and qPCR analyses ( Fig. 5a ) ( Supplementary Fig. S2 ). These data suggested that RORβ1 acts upstream of Ptf1a but in parallel with Foxn4 at early stages of amacrine and horizontal cell differentiation. The Ptf1a gene contains an RORβ1-responsive enhancer The mechanism of regulation of Ptf1a expression in the retina is unknown. Thus, loss of Ptf1a expression in 1g/1g mice suggested the hypothesis that RORβ1 induces the Ptf1a gene. Given that Foxn4 −/− mice similarly lacked Ptf1a expression [10] , we also tested whether RORβ1 and Foxn4 cooperatively induced Ptf1a . Previous studies identified a 2.2-kb upstream region and a 12.4-kb downstream region of the Ptf1a gene that directed reporter transgene expression in the spinal cord, hindbrain, pancreas and retina in mice [33] , [34] . We tested conserved fragments from these regions for enhancer function in response to RORβ1 and Foxn4 using a luciferase reporter with a 0.6-kb Ptf1a promoter region ( Fig. 6a ). When transfected into 293 T cells, a 1.6-kb downstream fragment, or a 0.8-kb sub-domain of this fragment (En0.8), conferred a remarkable ≥90 fold synergistic activation of the reporter in the presence of both RORβ1 and Foxn4 when normalized over basal expression in the absence of added factors ( P <0.001). In contrast, RORβ1 and Foxn4 individually gave only 3.3-fold and 5.1-fold activation, respectively ( Fig. 6c ) (difference for both factors compared with RORβ1 alone P <0.001, or Foxn4 alone P <0.001). In comparison, other enhancer fragments tested, including the upstream 2.2 kb fragment (Pr/En2.2) gave relatively little change in the response to both factors compared with the promoter alone reporter. 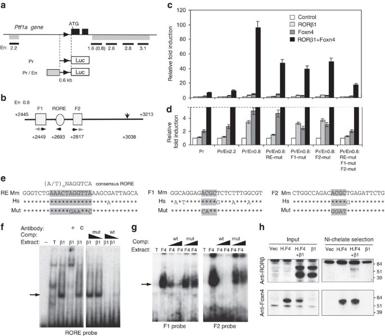Figure 6: RORβ1-responsive enhancer inPtf1agene. (a)Ptf1agene; black boxes, exons; triangle, promoter; grey bars below gene, enhancer regions. Enhancer (En) fragments tested are shown as black bars with size (kb) below. Reporter constructs contained a 0.6-kbPtf1apromoter driving luciferase without (Pr) or with enhancer fragments (Pr/En). (b) Foxn4 (F1, F2) and RORβ1 (RORE) response elements in En0.8 fragment. Arrowheads, motifs and orientation; black arrowheads, conserved between mouse and human genomes. Numbers, distances (in bp) from ATG. Vertical arrow (+3038) indicates a distant control mutation. (c) Luciferase assays in 293T cells for reporter responses to RORβ1 and Foxn4 normalized to basal expression of each reporter in absence of added factors; means±s.d. Pr/En0.8 gave >10-fold greater synergistic induction than Pr promoter alone (P<0.001). Fold induction of Pr/En0.8 by both factors together (black columns) was reduced by individual or combined mutagenesis (mut) of RORE, F1 and F2 sites (P<0.001 for each mutant compared with wild-type). Statistical analyses were performed using Student’st-test. (d) Magnification of lower region of response scale in panel ‘c’.Note:responses to both factors (black columns) are truncated above the dashed line. (e) RORE, F1 and F2 sequences in mouse (Mm) and human (Hs) genomes; asterisks indicate identity; core motifs shaded. Mouse wild-type and mutant (mut) sequences were used as EMSA probes. (f) EMSA of RORβ1 binding to RORE using extracts from 293T cells transfected with RORβ1-expressing (β1) or empty (T) vector; probe alone (−). Competition with wild-type (wt) but not mutant (mut) unlabelled oligonucleotides abolished the shifted band (arrow). Anti-RORβ antibody (+) but not IgG control (c) supershifted the band. (g) EMSA of Foxn4 binding to F1 and F2 using extracts from 293T cells transfected with Foxn4-expressing (F4) or empty (T) vector. Competition with wild-type but not mutant oligonucleotides strongly diminished the shifted band (arrow). (h) Protein interaction between RORβ1 and Foxn4. Left, input protein from 293T cells transfected with empty vector (vec), or vectors expressing histidine-tagged Foxn4 (H.F4), RORβ1 (β1) or both (H.F4+β1) analysed by western blot (RORβ, upper; Foxn4, lower). Right, Nickel-chelate selection for H.F4 protein co-selected a weak RORβ1 band. Protein molecular size marker, kDa. Figure 6: RORβ1-responsive enhancer in Ptf1a gene. ( a ) Ptf1a gene; black boxes, exons; triangle, promoter; grey bars below gene, enhancer regions. Enhancer (En) fragments tested are shown as black bars with size (kb) below. Reporter constructs contained a 0.6-kb Ptf1a promoter driving luciferase without (Pr) or with enhancer fragments (Pr/En). ( b ) Foxn4 (F1, F2) and RORβ1 (RORE) response elements in En0.8 fragment. Arrowheads, motifs and orientation; black arrowheads, conserved between mouse and human genomes. Numbers, distances (in bp) from ATG. Vertical arrow (+3038) indicates a distant control mutation. ( c ) Luciferase assays in 293T cells for reporter responses to RORβ1 and Foxn4 normalized to basal expression of each reporter in absence of added factors; means±s.d. Pr/En0.8 gave >10-fold greater synergistic induction than Pr promoter alone ( P <0.001). Fold induction of Pr/En0.8 by both factors together (black columns) was reduced by individual or combined mutagenesis (mut) of RORE, F1 and F2 sites ( P <0.001 for each mutant compared with wild-type). Statistical analyses were performed using Student’s t -test. ( d ) Magnification of lower region of response scale in panel ‘c’. Note: responses to both factors (black columns) are truncated above the dashed line. ( e ) RORE, F1 and F2 sequences in mouse (Mm) and human (Hs) genomes; asterisks indicate identity; core motifs shaded. Mouse wild-type and mutant (mut) sequences were used as EMSA probes. ( f ) EMSA of RORβ1 binding to RORE using extracts from 293T cells transfected with RORβ1-expressing (β1) or empty (T) vector; probe alone (−). Competition with wild-type (wt) but not mutant (mut) unlabelled oligonucleotides abolished the shifted band (arrow). Anti-RORβ antibody (+) but not IgG control (c) supershifted the band. ( g ) EMSA of Foxn4 binding to F1 and F2 using extracts from 293T cells transfected with Foxn4-expressing (F4) or empty (T) vector. Competition with wild-type but not mutant oligonucleotides strongly diminished the shifted band (arrow). ( h ) Protein interaction between RORβ1 and Foxn4. Left, input protein from 293T cells transfected with empty vector (vec), or vectors expressing histidine-tagged Foxn4 (H.F4), RORβ1 (β1) or both (H.F4+β1) analysed by western blot (RORβ, upper; Foxn4, lower). Right, Nickel-chelate selection for H.F4 protein co-selected a weak RORβ1 band. Protein molecular size marker, kDa. Full size image The 0.8 kb sub-fragment contained a candidate RORβ1 response element (RORE, 5′-AAACTAGGTTA-3′) related to the 5′-(A/T) n NAGGTCA-3′ consensus [29] , [27] ( Fig. 6b ). This RORE was 100% conserved and the surrounding 760 bp sequence was 75% conserved between human and mouse genomes. Mutagenesis of the RORE in the context of En0.8 impaired both the individual response to RORβ1 and the synergistic response to RORβ1 and Foxn4 (each P <0.001 compared with wild-type Pr/En0.8) ( Fig. 6c ). A control mutation 345 bp distant from the RORE interfered minimally with responses to RORβ1 and Foxn4 (not shown). En0.8 also contained two putative elements for Foxn factors based on a core ACGC motif [35] , [32] , located 185 bp upstream (F1) and 125 bp downstream (F2) of the RORE ( Fig. 6b ). Of two candidate ACGC motifs in F1, the downstream site and flanking bases were conserved in mouse and human genomes, whereas in F2, the most upstream of two candidate motifs was conserved. Individual mutagenesis of ACGC motifs in F1 and in F2 partly reduced the synergistic response to RORβ1 and Foxn4 ( P <0.001), whereas combined mutagenesis of RORE, F1 and F2 more severely diminished the response ( P <0.001) ( Fig. 6c ). Direct regulation of the Ptf1a gene by RORβ1 and Foxn4 was suggested by DNA-binding studies. In an electrophoretic mobility shift assay (EMSA), an oligonucleotide probe representing the RORE in the En0.8 enhancer bound RORβ1 protein obtained by overexpression in 293T cells ( Fig. 6f ). The shifted band was diminished by addition of excess wild-type but not mutant competitor oligonucleotides. The shifted band was also supershifted by addition of antibody against RORβ but not by a control immunoglobulin. Also, probes containing the conserved ACGC sequences in F1 and F2 each bound Foxn4 protein in EMSA ( Fig. 6g ). The specific shifted band for each probe was diminished strongly by wild-type but weakly by mutant competitor oligonucleotides. Although the molecular basis of the synergy between RORβ1 and Foxn4 remains unclear, the possibility that RORβ1 and Foxn4 interact physically was investigated by protein pull-down analyses using extracts from 293T cells that overexpress RORβ1 (β1) and histidine-tagged Foxn4 (H.F4) ( Fig. 6h ). Isolation of tagged Foxn4 by nickel-chelate chromatography co-selected RORβ1, which was identified by western blot analysis. The co-selected RORβ1 band was specific but relatively weak. However, in EMSA, the addition of both Foxn4 and RORβ1 did not alter the migration of the RORE probe compared with the shift given by RORβ1 alone, indicating that the RORE site did not represent a composite element that bound a dimeric RORβ1/Foxn4 protein complex (not shown). A reciprocal experiment also indicated that F1 or F2 probes did not represent composite DNA-binding sites for RORβ1/Foxn4 complexes. The evidence suggests that RORβ1 and Foxn4 primarily bind to their respective DNA elements in the Ptf1a gene and only secondarily contact each other. RORβ1 promotes amacrine cell generation To determine if RORβ1 stimulates differentiation in a gain-of-function experiment, a vector expressing RORβ1 from a constitutively active ubiquitin promoter (Ub/RORβ1) was electroporated into the retina of neonatal (P0) mice [36] ( Fig. 7 ). A co-electroporated plasmid expressing Td tomato (TdT) allowed identification of electroporated cells. Differentiation outcomes were analysed at P14, when amacrine and horizontal cell populations normally have been formed and can be identified by their morphology and location in the retinal layers. 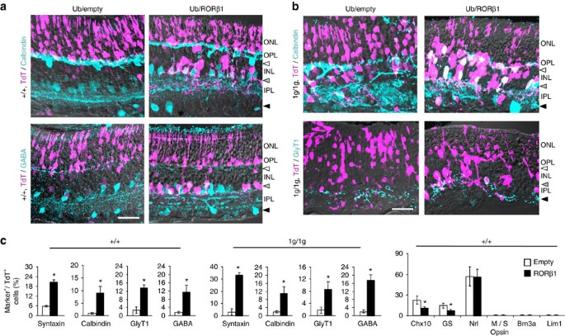Figure 7: RORβ1 promotes amacrine cell differentiation. (a) Retinal sections of +/+ mice at P14 after electroporation at P0 with Ub/empty control or Ub/RORβ1-expression vector. Electroporated cells were identified by co-electroporated TdT marker. TdT+(purple), calbindin+or GABA+amacrine cells (turquoise) and double-positive cells (white/whitish) were visualized by confocal imaging. Horizontal, amacrine and displaced amacrine cell zones are indicated by white, grey and black arrowheads, respectively. Ub/RORβ1 yielded many TdT+amacrine cells with projections in the inner plexiform layer. Scale bar, 30 μm in all panels. (b) In RORβ1-deficient (1g/1g) pups electroporated at P0 and analysed at P14, Ub/RORβ1 yielded many TdT+amacrine-like cells in the INL with projections in the inner plexiform layer. TdT+, calbindin+cells with unusual projections in the outer plexiform layer may be mis-located amacrine cells in the disorganized INL of 1g/1g mice. (c) Counts of cells positive for amacrine (syntaxin, GABA, GlyT1) and combined amacrine/horizontal (calbindin) markers in +/+ (left) and 1g/1g (middle) mice. Counts represent marker+/TdT+electroporated cells in 150 μm lengths of retina. Right, counts in +/+ mice of cells positive for TdT and bipolar (Chx10), Muller glial (glutamine synthetase, GS), rod (Nrl), cone (M and S opsin), ganglion (Brn3a) or horizontal (Lim1) cell markers. Means±s.d.; ≥6 eyes from ≥6 mice; *P<0.001. Statistical analyses were performed using Student’st-test. Figure 7: RORβ1 promotes amacrine cell differentiation. ( a ) Retinal sections of +/+ mice at P14 after electroporation at P0 with Ub/empty control or Ub/RORβ1-expression vector. Electroporated cells were identified by co-electroporated TdT marker. TdT + (purple), calbindin + or GABA + amacrine cells (turquoise) and double-positive cells (white/whitish) were visualized by confocal imaging. Horizontal, amacrine and displaced amacrine cell zones are indicated by white, grey and black arrowheads, respectively. Ub/RORβ1 yielded many TdT + amacrine cells with projections in the inner plexiform layer. Scale bar, 30 μm in all panels. ( b ) In RORβ1-deficient (1g/1g) pups electroporated at P0 and analysed at P14, Ub/RORβ1 yielded many TdT + amacrine-like cells in the INL with projections in the inner plexiform layer. TdT + , calbindin + cells with unusual projections in the outer plexiform layer may be mis-located amacrine cells in the disorganized INL of 1g/1g mice. ( c ) Counts of cells positive for amacrine (syntaxin, GABA, GlyT1) and combined amacrine/horizontal (calbindin) markers in +/+ (left) and 1g/1g (middle) mice. Counts represent marker + /TdT + electroporated cells in 150 μm lengths of retina. Right, counts in +/+ mice of cells positive for TdT and bipolar (Chx10), Muller glial (glutamine synthetase, GS), rod (Nrl), cone (M and S opsin), ganglion (Brn3a) or horizontal (Lim1) cell markers. Means±s.d. ; ≥6 eyes from ≥6 mice; * P <0.001. Statistical analyses were performed using Student’s t -test. Full size image Compared with Ub/empty vector, Ub/RORβ1 electroporated into +/+ mice of the CD1 strain yielded large numbers of TdT + cells in the amacrine cell zone of the INL with projections typical of amacrine cells in the inner plexiform layer. Many of these TdT + cells also expressed markers for amacrine cell types (GABA, calbindin, GlyT1, syntaxin) ( Fig. 7a ). However, Ub/RORβ1 yielded few detectable cells in the location of horizontal cells or displaced amacrine cells, probably reflecting limited competence of progenitor cells at the neonatal stage to form some cell types because horizontal cells and a large proportion of amacrine cells have normally been formed by P0 [3] , [5] . Apart from increased amacrine cell numbers, Ub/RORβ1 gave diminished numbers of Chx10 + bipolar cells and glutamine synthetase + Müller glial cells compared with Ub/empty vector ( Fig. 7c ), suggesting that ectopic expression of RORβ1 may inhibit progenitors at P0 from acquiring certain cell fates. Analysis of markers for rods (Nrl), cones (M and S opsin), ganglion cells (Brn3a) and horizontal cells (Lim1) revealed no differences in response to Ub/RORβ1 or Ub/empty vector. The lack of cells positive for cone, ganglion and horizontal cell markers was consistent with restricted competence of progenitors at P0 to form certain cell types. In summary, ectopic expression of RORβ1 at P0 stimulated amacrine cell differentiation and partly suppressed bipolar and Müller glial cell outcomes. We also investigated whether RORβ1 can rescue amacrine and horizontal cell differentiation in neonatal RORβ1-deficient mice ( Fig. 7b ). Compared with Ub/empty vector, Ub/RORβ1 yielded many TdT + amacrine-like cells, including syntaxin + , GABA + , GlyT1 + and calbindin + cells in the INL with projections in the inner plexiform layer in 1g/1g mice. Ub/RORβ1 also produced TdT + /calbindin + cells at the outer zone of the INL with lateral projections in the outer plexiform layer. Although these cells resided in the location of horizontal cells, they probably represented amacrine cells that had failed to align in the amacrine cell zones in the disorganized INL in 1g/1g mice, as horizontal cells are normally produced only during embryogenesis [4] . We also detected GABA, an amacrine cell marker, in TdT + cells at this location (not shown). In summary, ectopic overexpression studies indicate that RORβ1 promotes amacrine cell but not horizontal cell differentiation in +/+ or 1g/1g mice at P0. This study indicates that RORβ1 is critical for the differentiation of amacrine and horizontal cells and for the transcriptional induction of Ptf1a, a necessary factor for the generation of both of these classes of interneurons. The synergistic activation of the Ptf1a gene by RORβ1 with Foxn4 suggests that a novel cooperation between an orphan nuclear receptor and a forkhead box factor directs a transcriptional pathway for amacrine and horizontal cell differentiation. We propose a model in which RORβ1 and Foxn4 cooperatively prompt progenitors to commit to form precursors for horizontal and amacrine cell types ( Fig. 8 ). A requirement for two factors, rather than only one, may impose stringent selection over which progenitors make this commitment. Consequently, only the requisite cell population may become committed while adequate pools of progenitors are retained for the generation of other retinal cell types. Foxn4 is restricted to dividing progenitors [9] such that the immediate result of RORβ1 and Foxn4 cooperation may be induction of Ptf1a which is transiently expressed in post-mitotic precursor cells for both classes of interneurons [10] , [11] . In accord with this early role for RORβ1, Rorb 1g/1g mice have reduced expression of many later-acting transcription factors involved in terminal differentiation of horizontal and amacrine cell sub-lineages. Unlike Foxn4, RORβ1 continues to be expressed in post-mitotic horizontal and amacrine cells and may possibly also contribute to later maturational events. 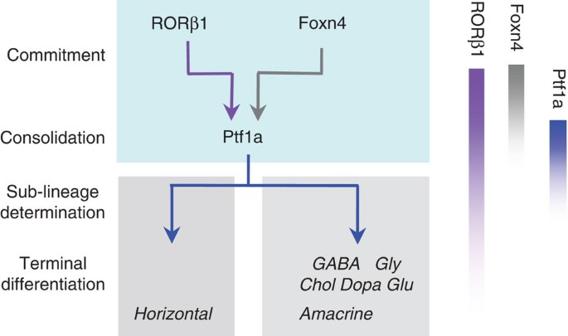Figure 8: Proposed role for RORβ1 in amacrine and horizontal cell differentiation. It is proposed that RORβ1 and Foxn4 in progenitor cells cooperatively promote commitment to amacrine and horizontal cell fates by synergistic induction of Ptf1a. Ptf1a is transiently induced in post-mitotic precursors and consolidates the fates of both classes of interneurons. Many factors (not shown) contribute to the subsequent terminal differentiation of horizontal and amacrine cell sub-lineages, indicated here according to main neurotransmitter types (GABA, glycine, acetyl choline, dopamine, glutamate). Relative timing of expression of RORβ1, Foxn4 and Ptf1a is indicated on the right: Foxn4 is in dividing progenitors, Ptf1a in post-mitotic precursors and RORβ1 in both progenitors and precursors. Figure 8: Proposed role for RORβ1 in amacrine and horizontal cell differentiation. It is proposed that RORβ1 and Foxn4 in progenitor cells cooperatively promote commitment to amacrine and horizontal cell fates by synergistic induction of Ptf1a. Ptf1a is transiently induced in post-mitotic precursors and consolidates the fates of both classes of interneurons. Many factors (not shown) contribute to the subsequent terminal differentiation of horizontal and amacrine cell sub-lineages, indicated here according to main neurotransmitter types (GABA, glycine, acetyl choline, dopamine, glutamate). Relative timing of expression of RORβ1, Foxn4 and Ptf1a is indicated on the right: Foxn4 is in dividing progenitors, Ptf1a in post-mitotic precursors and RORβ1 in both progenitors and precursors. Full size image Deficiency of either RORβ1 or Foxn4 [9] results in a partial reduction of expression of Nd1 and Nd4, which are required for amacrine but not horizontal cell differentiation [15] . Thus, RORβ1 and Foxn4 may reside upstream of Nd1 and Nd4, although quantification of Nd1 and Nd4 expression in the pertinent cells is difficult to accomplish as these factors are expressed in many retinal cell types in developmentally changing patterns. Conceivably, in amacrine cell differentiation, Nd1 and Nd4 act upstream of, or in parallel with, Ptf1a because Nd1 and Nd4 expression is unperturbed in Ptf1a −/− mice [10] , [11] . A given transcription factor gene may control diverse neurodevelopmental functions although the basis for this versatility is often unclear. Our evidence indicates that for Rorb , such versatility is facilitated by two properties: first, the ability of RORβ proteins to cooperate with other cell-specific factors, such as Foxn4, and second, the ability of the gene to express distinct RORβ1 and RORβ2 isoforms in cell-specific patterns. RORβ isoforms possess specific DNA-binding properties but only weak trans-activating functions, such that cooperation with other activators in different cell types can allow the induction of specific target genes. Cooperation between RORβ1 and Foxn4 produces a potent synergistic induction of Ptf1a expression. Although the mechanism is unclear at present, the evidence indicates that RORβ1 and Foxn4 each bind to distinct sites within a 350-bp enhancer region in the Ptf1a gene. Potentially, the coordinated binding of both factors leads to recruitment of other co-activators or chromatin-activating complexes that stimulate the promoter of the gene. RORβ isoforms also cooperate with Crx homeodomain factor to induce the Opn1sw opsin gene in cones [27] and probably also with Otx2 homeodomain factor to induce the Nrl gene in rods [28] , [37] , [38] . In each case, DNA-binding sites exist for both the RORβ isoform and its cooperating factor suggesting that DNA binding by both factors is required for transcriptional enhancement. Cooperative interactions have also been suggested to allow regulation of the activity of orphan receptors that lack known physiological ligands. For example, DNA-binding activity by Drosophila Ftzf1 nuclear receptor is regulated by interaction with a homeodomain protein [39] . The differential expression of N-terminal variant isoforms provides a precise means by which a nuclear receptor gene can direct distinct cellular functions. Thus, RORβ1 mediates differentiation of amacrine and horizontal cells and also control of hindlimb movement. The function of the RORβ2 isoform is currently undefined but the contrasting expression profiles of RORβ1 and RORβ2, and the differing phenotypes of mice deleted for RORβ1 or all RORβ isoforms, implicate RORβ2 in photoreceptor differentiation [26] , [27] , [28] . Highly specialized, cell-specific functions have also been described for isoforms encoded by the retinoid-related orphan receptor γ ( Rorg ) and thyroid hormone receptor β ( Thrb ) genes. The RORγt isoform encoded by Rorg serves critical functions in inflammatory lymphoid cells [40] , whereas the TRβ2 isoform encoded by Thrb controls a key step in the differentiation of cone photoreceptors [41] . Targeted mutagenesis and retinal electroporation RORβ1 and RORβ2-specific exons were identified by alignment of mouse genomic and cDNA sequences (accession nos. NM_001043354, NM_146095). Genomic Rorb 5′ and 3′ homology arms isolated from ES cell DNA using Phusion polymerase (NewEngland Biolabs) were inserted into a pACN vector carrying a self-excisable neomycin-resistance gene ( tACE-Cre-Neo ) [42] . An enhanced gfp cDNA replaced the RORβ1-specific exon. Targeted W9.5 ES cell clones were used to generate chimeric mice by K. Kelley at the Genetics Core Facility, Mount Sinai School of Medicine. Chimeras were crossed with C57BL/6J mice, then Rorb +/1g mice intercrossed to generate +/+, +/1g and 1g/1g progeny on a C57BL/6J x 129/Sv background for analysis. The ACN cassette self-excised during germline transmission from male chimeras to yield the Rorb 1g allele. Genotypes were determined by Southern blot or PCR using as primers: common reverse 5′-GCCTCTTCTACCCAAAGTCAC-3′, wild-type forward 5′-TCATGCGAGGTAAGCGAGC-3′, mutant forward 5′-CAACTACAACAGCCACAACG-3′, yielding wild-type and mutant bands of 358 and 653 bp, respectively. In vivo electroporation was performed as described [36] in wild-type CD1 or Rorb 1 g/1g pups on the mixed background noted above. RORβ1 and Foxn4 cDNAs were inserted into a Ub expression vector [43] . Animal experiments were performed in accordance with protocols approved by the Animal Care and Use Committee at NIDDK and NEI at the National Institutes of Health. qPCR and western blot analysis RNA from pooled retinas (>4 mice per pool) was subjected to reverse transcription and real-time qPCR with normalization to β-actin mRNA levels [28] using primers for Foxn4, Ptf1a, Nd1 Nd4, Lim1, Brn3b, Barhl2, Ebf3, bHLHb5 and Nr4a2 ( Supplementary Table S2 ). Developmental analysis of RORβ1 and RORβ2 mRNA levels ( Fig. 1a ) was determined in triplicate on retinal RNA samples pooled from >3 mice at each age using primers as follows: β1F, 5′-CCATCAGAAACAGTCATCAGCAAC-3′, β1R 5′-TGGGCAGGAGTAAGAGGCATTG-3′, β2F, 5′-CCGTCAGAATGTGTGAGAACCAG-3′, β2R 5′-ATCCTCCCGAACTTTACAGCATC-3′. Samples represented dissected retina except at E13.5, at which age whole eye was used. Western blot analysis was performed on 10 or 20 μg samples of retinal proteins using antibodies for RORβ (rabbit polyclonal, 1/1000, Diagenode pAbRORbHS100) and actin (mouse monoclonal, 1/5000, Millipore MAb1501) with chemiluminescent detection [44] . In situ hybridization and immunohistochemistry Digoxigenin-labelled antisense and sense riboprobes were used for in situ hybridization on 10 μm retinal cryosections with colorigenic detection as described [44] . For immunostaining, 10 μm cryosections were incubated overnight with primary antibody at 4 °C, then incubated with fluorescent-conjugated second antibody for 1 h at room temperature, gently washed three times in 1xPBS before addition of mounting medium. Antibodies and dilutions are listed in Supplementary Table S1 . Double analysis for gfp and PCNA (or BrdU) required pre-treatment of sections in 2 M HCl at room temperature for 10 min, followed by neutralization in 0.1 M sodium borate buffer for 10 min before addition of antibody against PCNA or BrdU. For flatmounts, the eye was fixed in 4% PFA at 4 °C for 1 h. The cornea, lens and pigmented epithelium were removed, then the retinal cup incubated with antibody in blocking buffer for 2–3 days at 4 °C, washed several times in PBS for 6 h, then incubated with second fluorescent antibody for 1 day. The retina was washed in PBS for 2 h, cut peripherally with 3–5 incisions then flattened on a slide. For BrdU labelling, pregnant female mice or neonatal pups were injected intraperitoneally with 20 μg BrdU/g weight from a 10-μg/μl stock solution 1 h before eye dissection. For immunofluorescence, a Leica laser scanning confocal microscope analysed 0.5 μm planar images stacked to a total 4 μm thickness for retinal flatmounts or sections of electroporated retinas, or a single 0.5 μm plane for other sections. Image brightness and contrast were adjusted using ImageJ (NIH, Bethesda, MD). Cell count data represent means±s.d. Statistical analyses of cell counts were performed using Student’s two-tailed t -test to compare 1g/1g versus +/+ samples, or test versus control samples in electroporation experiments. For histology, 3 μm methacrylate plastic sections near the vertical mid-line of the eye were stained with hematoxylin and eosin [44] . Reporter plasmid constructs and luciferase assays Ptf1a promoter and enhancer fragments from C57BL/6J mouse DNA were inserted into pREP4 luciferase reporter vector. Mutations were introduced by site-directed mutagenesis into the reporter vectors using oligonucleotides to change the RORE, F1 and F2 Foxn response elements as follows (changed bases in bold and italics within the underlined core motifs): RORE-mutation 5′-GGGTCTGAAACT GAA TT C AAGCGATTAGCA-3′; F1 mutation 5′-GA GC TA GGGGTTGGGGCAGGAG CA GC TC-3′; F2 mutation 5′-AC GGAT TGAGATTCTGGGTCGCG T CGC TC-3′. Note that for F1 and F2 elements, both candidate Foxn response motifs (ACGC) were changed in each element. Mouse RORβ1 and Foxn4 cDNAs were expressed from pSG5 or pCDNA3.1 vectors transfected into 293T cells in 24-well plates in mixtures containing 100 ng reporter, 5 ng pSV-RL renilla control plasmid, 400 ng expression plasmid and carrier DNA to a total of 800 ng DNA with 2 μl Fugene HD reagent (Roche). Luciferase activity was measured 48 h after transfection. Samples were analysed in triplicate and each experiment was repeated three times. Data represent mean±s.d. Statistical analysis was performed by Student’s t -test under different categories: (i) basal activity of each reporter in the absence of added factors was compared individually with promoter alone (Pr) reporter, to rule out basal variations that could distort subsequent analyses of induction; none was significantly different from Pr alone ( P >0.26); (ii) for determination of the synergistic response of each reporter, the normalized fold induction in the presence of both RORβ1 and Foxn4 was compared with that in the absence of factors or in the presence of only RORβ1 or Foxn4; (iii) to determine the activity of each enhancer fragment, the fold induction of each reporter in the presence of both factors was compared with that of promoter alone (Pr) in the presence of both factors; (iv) to assess the result of mutagenesis of RORE, F1 or F2 in the context of Pr/En0.8, the fold induction over basal level of each mutation construct in the presence of RORβ1 and Foxn4 was compared with the fold induction of wild-type Pr/En0.8 in the presence of RORβ1 and Foxn4. EMSA and protein co-selection analyses EMSA was performed with 2 μg of nuclear protein extract from transfected 293T cells and 0.2 pmol of [32] [P] end-labelled probe as described [27] . Antibody against RORβ or control IgG was pre-incubated with protein at 4 °C for 30 min before addition of probe, then incubated at room temperature for 15 min. Competitor probe was added at 5- or 50-fold excess. For protein pull-down studies, extracts from 293T cells transfected with RORβ1 and His 6 -Foxn4 expression plasmids were incubated with Ni-beads for 2 h at 4 °C ( [27] ). The histidine tag was fused onto the C-terminus of Foxn4. Proteins were released by heating at 95 °C then analysed by electrophoresis and western blot. How to cite this article: Liu, H. et al . An isoform of retinoid-related orphan receptor β directs differentiation of retinal amacrine and horizontal interneurons. Nat. Commun. 4:1813 doi: 10.1038/ncomms2793 (2013).